New class of nonaqueous electrolytes for long-life and safe lithium-ion batteries Long-life and safe lithium-ion batteries have been long pursued to enable electrification of the transportation system and for grid applications. However, the poor safety characteristics of lithium-ion batteries have been the major bottleneck for the widespread deployment of this promising technology. Here, we report a novel nonaqueous Li 2 B 12 F 12- x H x electrolyte, using lithium difluoro(oxalato)borate as an electrolyte additive, that has superior performance to the conventional LiPF 6 -based electrolyte with regard to cycle life and safety, including tolerance to both overcharge and thermal abuse. Cells tested with the Li 2 B 12 F 9 H 3 -based electrolyte maintained about 70% initial capacity when cycled at 55 °C for 1,200 cycles, and the intrinsic overcharge protection mechanism was active up to 450 overcharge abuse cycles. Results from in situ high-energy X-ray diffraction showed that the thermal decomposition of the delithiated Li 1- x [Ni 1/3 Mn 1/3 Co 1/3 ] 0.9 O 2 cathode was delayed by about 20 °C when using the Li 2 B 12 F 12 -based electrolyte. Since the commercialization of the lithium-ion battery by Sony Corporation in the early 1990s, the capacity of a single 18,650 lithium-ion cell, which is 65 mm in height and 18 mm in diameter, has been tripled. The dramatic increase in capacity was mainly achieved through changes in the engineering design to load more active materials into the cell, as well as the development of battery materials and processes that allow a wider operational potential window. For example, LiCoO 2 is the conventional cathode material and generally delivers a specific capacity of about 148 mAh g −1 by limiting the cutoff potential to 4.2 V versus Li + /Li, while advanced cathode materials can deliver more than 200 mAh g −1 by raising their working potential [1] , [2] , [3] . While the physical and electrochemical boundaries of lithium-ion batteries have been and continue to be aggressively pushed to achieve higher energy density, their intrinsic safety has emerged as a primary technological barrier for the transportation application [4] , [5] . Recent efforts to address the safety issue of lithium-ion batteries include development of electrolyte additives to improve the thermal stability of lithiated anodes [6] , [7] and surface coatings for cathode materials to provide physical protection between the charged electrodes and the electrolyte [8] , [9] . The underlying premise behind these approaches directly or indirectly relates to the thermal/chemical instability of the LiPF 6 electrolyte, which tends to generate hydrofluoric (HF) acid when exposed to a trace amount of moisture. The HF accelerates the corrosion of cathode materials (lithium transition metal oxides) and the migration of transition metal-based compounds from the cathode to the graphitic anode [10] , a process that compromises the thermal stability of the solid electrolyte interphase (SEI), which is critical to protecting the graphitic anode from attack by the electrolyte [6] . In addition, protons have been reported to intercalate into delithiated lithium transition metal oxide cathodes and thereby reduce the chemical stability of the delithiated cathodes [11] , [12] . Here, we demonstrate that these shortcomings mentioned above can be resolved by replacing LiPF 6 with an alternative lithium salt, such as Li 2 B 12 F 12- x H x . Lithium-ion cells using Li 2 B 12 F 12- x H x -based electrolytes with proper additives to form stable SEI layer on graphitic anode maintained about 70% initial capacity after cycling at 55 °C for 1,200 cycles. In addition, these cells also showed outstanding intrinsic tolerance towards both continuous and pulse overcharge abuse. In situ high-energy X-ray diffraction (HEXRD) study indicated that the delithiated Li 1- x [Ni 1/3 Mn 1/3 Co 1/3 ] 0.9 O 2 with the presence of Li 2 B 12 F 9- x F x -based electrolytes had a better thermal stability than those with the presence of LiPF 6 -based electrolytes. Electrochemical activity of Li 2 B 12 F 12- x H x Unlike LiPF 6 , Li 2 B 12 F 12- x H x salts are compatible with a high concentration of water in the electrolyte. When a high concentration of water, up to 10,000 ppm, was added to the LiPF 6 -based electrolyte, the water was quickly consumed by reaction with LiPF 6 and generated a high concentration of HF in the electrolyte ( Fig. 1 ). However, the water concentration did not change in the Li 2 B 12 F 9 H 3 -based electrolyte, and no HF was detected up to 10 days at room temperature, even with the presence of 35,000 ppm water. In addition, Li 2 B 12 F 12- x H x salts have a unique redox shuttle capability that can provide overcharge protection and automatic capacity balancing of lithium-ion cells when present in a battery pack ( Fig. 2 ). 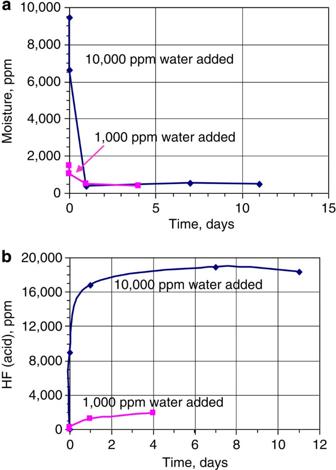Figure 1: Reaction of LiPF6with water presented in the electrolyte. Detected moisture level (a) and HF (b) in the 1.0 M LiPF6in EC/EMC with a ratio of 1:1 by weight after the addition of 1,000 ppm (pink) and 10,000 ppm water (blue). Figure 1: Reaction of LiPF 6 with water presented in the electrolyte. Detected moisture level ( a ) and HF ( b ) in the 1.0 M LiPF 6 in EC/EMC with a ratio of 1:1 by weight after the addition of 1,000 ppm (pink) and 10,000 ppm water (blue). 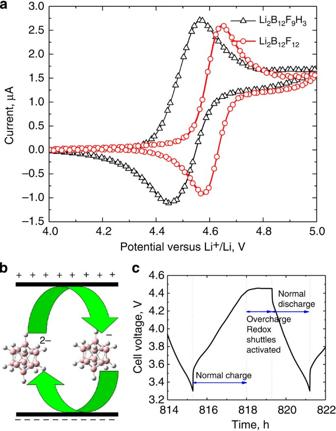Figure 2: Reversible redox reaction of B12F122−and B12F9H32−for overcharge protection of lithium-ion cells. (a) Cyclic voltammograms of 10 mM Li2B12F9H3and Li2B12F12in 1.2 M LiPF6in EC/EMC using a Pt/Li/Li three-electrode cell at a scanning rate of 10 mV s−1. (b) Schematic of overcharge protection mechanism provided by the salts. (c) Voltage profile of mesocarbon microbeads/Li1.1[Ni1/3Mn1/3Co1/3]0.9O2cell during overcharge test showing the positive effect of Li2B12F9H3. Full size image Figure 2: Reversible redox reaction of B 12 F 12 2− and B 12 F 9 H 3 2− for overcharge protection of lithium-ion cells. ( a ) Cyclic voltammograms of 10 mM Li 2 B 12 F 9 H 3 and Li 2 B 12 F 12 in 1.2 M LiPF 6 in EC/EMC using a Pt/Li/Li three-electrode cell at a scanning rate of 10 mV s −1 . ( b ) Schematic of overcharge protection mechanism provided by the salts. ( c ) Voltage profile of mesocarbon microbeads/Li 1.1 [Ni 1/3 Mn 1/3 Co 1/3 ] 0.9 O 2 cell during overcharge test showing the positive effect of Li 2 B 12 F 9 H 3 . Full size image The cyclic voltammograms in Fig. 2a show that both Li 2 B 12 F 9 H 3 and Li 2 B 12 F 12 undergo a reversible redox reaction at 4.5 V and 4.6 V versus Li + /Li, respectively, both of which are high enough to provide overcharge protection to 4-V class cathode materials for lithium-ion batteries. However, Li 2 B 12 F 9 H 3 is preferred because less heat is generated during overcharge abuse, whose importance will be detailed later. Figure 2b illustrate the shuttle mechanism of the anion B 12 F 9 H 3 2− . During normal charge, when the potential of the cathode is lower than that of the B 12 F 9 H 3 2− redox shuttle, the anion remains inactive. When the cell is overcharged, the potential of the cathode reaches the redox potential of B 12 F 9 H 3 2− and its shuttle mechanism is then activated, during which B 12 F 9 H 3 2− is oxidized (losing an electron) at the cathode and diffuses back to the anode to be reduced (that is, gain an electron from the anode). According to this mechanism, the overcharge current can be shuttled through the lithium-ion cell without further increasing the cell voltage. Structure of B 12 F 12- x F x 2− /B 12 F 12- x F x − anions Ab initio calculations indicated that the B 12 F 12 2− anion has D 5 symmetry, and the lengths for the B-B and B-F bonds are 1.80 and 1.38 Å, respectively ( Supplementary Fig. S1 and Supplementary Table S1 ). When the anion is oxidized to form B 12 F 12 − , the D 5 symmetry is still maintained, with the B-B bond length extended to 1.88 Å, while the B-F bond length shrank to 1.34 Å to facilitate the donation of a lone electron pair on fluoride to the boron cage, helping to compensate for the loss of an electron during oxidation ( Supplementary Table S2 ). When some of the fluoride is replaced with hydrogen, the D 5 symmetry is broken for both the reduced and oxidized states. The structural change of B 12 F 9 H 3 2− during oxidation is similar to that of B 12 F 12 2− , although much smaller change was observed for B centres connected to H, as it has no lone electron pair for donating to the boron cage. 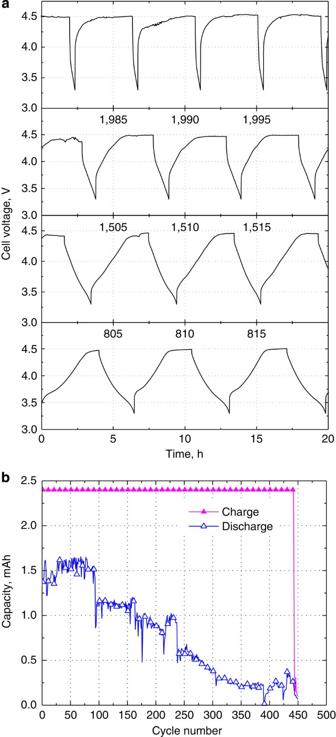Figure 3: Intrinsic overcharge protection of lithium-ion cells using Li2B12F9H3-based electrolyte. (a) Voltage profile of a graphite/Li1.1[Ni1/3Mn1/3Co1/3]0.9O2cell during continuous overcharge test at low rate (~C/3, 0.6 mA). The electrolytes consisted of 0.4 M Li2B12F9H3and 0.1 M LiBOB in EC/EMC, with additive of 1 wt% 2-(pentafluorophenyl)-tetrafluoro-1,3,2-benzodioxaborole. (b) Charge and discharge capacity of the cell shown inFig. 2aas function of cycle number. Intrinsic tolerance towards overcharge abuse Figure 3a shows the voltage profile of a graphite/Li 1.1 [Ni 1/3 Mn 1/3 Co 1/3 ] 0.9 O 2 lithium-ion cell during an overcharge abuse test (see Methods). The electrolyte was 0.4 M Li 2 B 12 F 9 H 3 and 0.1 M lithium bis(oxalato)borate (LiBOB) in a solvent of ethylene carbonate (EC) and ethyl methyl carbonate (EMC) with a ratio of 3:7 by weight; 1.0 wt% of 2-(pentafluorophenyl)-tetrafluoro-1,3,2-benzodioxaborole (PFPTFBB) was added as an electrolyte supplement. The charge/discharge capacity of the cell as a function of overcharge abuse cycle is shown in Fig. 3b . The graphite/Li 1.1 [Ni 1/3 Mn 1/3 Co 1/3 ] 0.9 O 2 cell had an initial reversible capacity of about 1.6 mAh. Figure 3: Intrinsic overcharge protection of lithium-ion cells using Li 2 B 12 F 9 H 3 -based electrolyte. ( a ) Voltage profile of a graphite/Li 1.1 [Ni 1/3 Mn 1/3 Co 1/3 ] 0.9 O 2 cell during continuous overcharge test at low rate (~C/3, 0.6 mA). The electrolytes consisted of 0.4 M Li 2 B 12 F 9 H 3 and 0.1 M LiBOB in EC/EMC, with additive of 1 wt% 2-(pentafluorophenyl)-tetrafluoro-1,3,2-benzodioxaborole. ( b ) Charge and discharge capacity of the cell shown in Fig. 2a as function of cycle number. Full size image During the overcharge abuse test, the cell was charged for 4 h with a constant current of 0.6 mA (~C/3) before being constant-current discharged to 3.0 V at 0.6 mA (~C/3). Figure 3a shows that the voltage of the cell was capped at about 4.5 V when B 12 F 9 H 3 2− was activated, and this overcharge protection mechanism was maintained up to about 450 cycles (2,000 h), even though the discharge capacity of the cell declined with the cycle number ( Fig. 3b ). The capacity degradation was attributed to either (1) the continuous growth of the interfacial impedance of the cell [13] or (2) accelerated cathode degradation when the cell was cycled up to 4.5 V versus Li + /Li (ref. 14 ). Most importantly, this superior overcharge tolerance was only obtained for the electrolyte containing additives of both LiBOB and PFPTFBB ( Supplementary Fig. S2 shows much inferior performance of cells without PFPTFBB). LiBOB is known to form a robust artificial SEI layer on the surface of graphite, which suppresses the reaction between lithiated graphite and the electrolyte [15] . With the presence of a Lewis acid such as PF 5 , LiBOB has a tendency to react with LiPF 6 to generate lithium difluoro(oxalato)borate (LiDFOB) and lithium tetrafluoro(oxalato)phosphate (LiTFOP) [16] ; both of these electrolyte additives have been reported to protect graphitic anodes [17] , [18] . We believe that a high concentration of Lewis acid (PFPTFBB [19] ) generates more LiDFOB or LiTFOP to maximize the protection for the graphitic anode. Therefore, LiDFOB was directly used as the electrolyte additive in place of LiBOB/ PFPTFBB in the following study. Graphite/Li 1.1 [Ni 1/3 Mn 1/3 Co 1/3 ] 0.9 O 2 lithium-ion chemistry has been long investigated as a promising candidate for the hybrid electric vehicle application, for which the battery is frequently pulse charged/discharged with high-rate current (up to 10 C) over short durations. Therefore, another cell was assembled and tested to evaluate its tolerance to repeated pulse overcharge abuse. The electrolyte was 0.4 M Li 2 B 12 F 9 H 3 in EC/EMC with 2.0 wt% LiDFOB as the electrolyte additive. After being constant-voltage charged to 4.1 V, the cell was overcharged for 100 pulses; in each pulse the cell was charged for 18 s with a constant current of 20 mA (~12 C) before resting for 1 h. A control cell using LiPF 6 -based electrolyte was tested by the same procedure, and the upper voltage of the cell quickly went beyond 4.9 V after only five pulses (compare Fig. 4a ). The voltage profile of the cell using Li 2 B 12 F 9 H 3 -based electrolytes during pulse overcharge is shown in Fig. 4b , demonstrating that the upper voltage was capped at 4.8 V during the pulse overcharge abuse test. 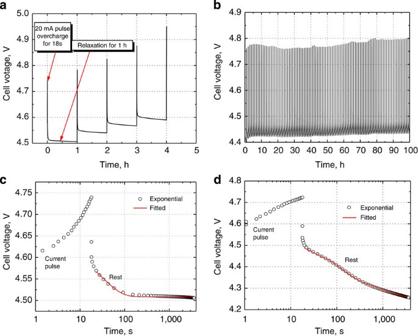Figure 4: High-rate pulse overcharge of lithium-ion cells. (a) Voltage profile of a graphite/Li1.1[Ni1/3Mn1/3Co1/3]0.9O2cell using LiPF6-based electrolyte during high-rate (~12 C, 20 mA) pulse overcharge. (b) Voltage profile of a graphite/Li1.1[Ni1/3Mn1/3Co1/3]0.9O2cell using Li2B12F9H3-based electrolyte during high-rate (~12 C, 20 mA) pulse overcharge. The electrolyte was 0.4 M Li2B12F9H3in EC/EMC (3:7, by weight) with 2.0 wt% LiDFOB as the electrolyte additive. (c) Fitting the typical voltage curve of LiPF6-based cells after pulse overcharge using an exponential decay function. (d) Fitting the typical voltage curve of Li2B12F9H3-based cells after pulse overcharge using an double exponential decay function. Figure 4c show the fitting results of voltage curves after the pulse overcharge using exponential decay functions for lithium-ion cells using LiPF 6 and Li 2 B 12 F 9 H 3 -based electrolytes, respectively. The fitting results in Fig. 4c used a single exponential decay function and indicate that the voltage relaxation was mostly caused by the relaxation of lithium-ion concentration after pulse charge. The voltage curve in Fig. 4d could only be fitted by a double exponential decay function, with one component representing the relaxation of lithium-ion concentration and the other representing the self-discharge of the over-delithiated cathode during the rest period, which was facilitated by the presence of shuttle mechanism between B 12 F 9 H 3 2− and B 12 F 9 H 3 − as shown in Fig. 2b . Figure 4: High-rate pulse overcharge of lithium-ion cells. ( a ) Voltage profile of a graphite/Li 1.1 [Ni 1/3 Mn 1/3 Co 1/3 ] 0.9 O 2 cell using LiPF 6 -based electrolyte during high-rate (~12 C, 20 mA) pulse overcharge. ( b ) Voltage profile of a graphite/Li 1.1 [Ni 1/3 Mn 1/3 Co 1/3 ] 0.9 O 2 cell using Li 2 B 12 F 9 H 3 -based electrolyte during high-rate (~12 C, 20 mA) pulse overcharge. The electrolyte was 0.4 M Li 2 B 12 F 9 H 3 in EC/EMC (3:7, by weight) with 2.0 wt% LiDFOB as the electrolyte additive. ( c ) Fitting the typical voltage curve of LiPF 6 -based cells after pulse overcharge using an exponential decay function. ( d ) Fitting the typical voltage curve of Li 2 B 12 F 9 H 3 -based cells after pulse overcharge using an double exponential decay function. Full size image Critic role of a stable SEI layer The long-term cycling performance was evaluated with graphite/Li 1.1 [Ni 1/3 Mn 1/3 Co 1/3 ] 0.9 O 2 pouch cells, whose initial reversible capacity was about 250 mAh. The electrolytes for these cells included (1) 1.2 M LiPF 6 in EC/EMC (3:7, by weight), (2) 1.2 M LiPF 6 in EC/EMC (3:7, by weight) with 2 wt% LiDFOB as the electrolyte additive, and (3) 0.4 M Li 2 B 12 F 9 H 3 in EC/EMC (3:7, by weight) with 2 wt% LiDFOB as the electrolyte additive. These cells were charged/discharged between 3.0 V and 4.1 V using a constant current of 80 mA (~C/3) at 55 °C. 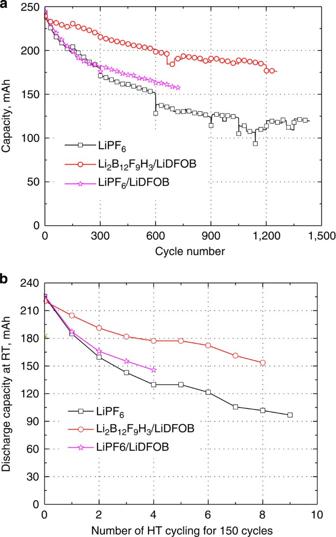Figure 5: Cycle life of lithium-ion cells using LiPF6-based and Li2B12F9H3-based electrolytes. (a) Discharge capacity as a function of cycle number for graphite/Li1.1[Ni1/3Mn1/3Co1/3]0.9O2lithium-ion cells cycled between 3.0 V and 4.1 V at a constant current of 0.5 mA (~C/3) at 55 °C. (b) Discharge capacity of graphite/Li1.1[Ni1/3Mn1/3Co1/3]0.9O2cells measured at room temperature. The cells are the same as those shown inFig. 5a; the capacity was measured at room temperature (RT) for every 150 cycles at 55 °C. Figure 5a shows the discharge capacity of the three pouch cells with different electrolytes cycled at 55 °C; the results indicate that the cell using Li 2 B 12 F 9 H 3 -based electrolyte had a much better capacity retention than the two using LiPF 6 -based electrolyte. The cell having Li 2 B 12 F 9 H 3 -based electrolyte maintained about 70% of initial reversible capacity after 1,200 cycles at 55 °C. Before and after every 150-cycle test at 55 °C, the cells were charged/discharged at room temperature over the same voltage range and at the same charge/discharge current for five cycles. Better capacity retention at room temperature was also obtained for the cell using the Li 2 B 12 F 9 H 3 -based electrolyte ( Fig. 5b ). Figure 5: Cycle life of lithium-ion cells using LiPF 6 -based and Li 2 B 12 F 9 H 3 -based electrolytes. ( a ) Discharge capacity as a function of cycle number for graphite/Li 1.1 [Ni 1/3 Mn 1/3 Co 1/3 ] 0.9 O 2 lithium-ion cells cycled between 3.0 V and 4.1 V at a constant current of 0.5 mA (~C/3) at 55 °C. ( b ) Discharge capacity of graphite/Li 1.1 [Ni 1/3 Mn 1/3 Co 1/3 ] 0.9 O 2 cells measured at room temperature. The cells are the same as those shown in Fig. 5a ; the capacity was measured at room temperature (RT) for every 150 cycles at 55 °C. Full size image A good SEI layer allows lithium ions to pass through while impeding the transportation of electrons, thereby suppressing the electrochemical reactions between the lithiated graphite and the electrolyte. Hence, an effective electrolyte additive such as LiBOB or LiDFOB can significantly improve the capacity retention of lithium-ion cells based on this mechanism ( Fig. 5 and Supplementary Fig. S3 ). What is unusual is that a stable/good SEI layer formed with LiBOB or LiDFOB and actually improved the overcharge protection capability of Li 2 B 12 F 9 H 3 ( Fig. 3 and Supplementary Fig. S2 ), although the redox shuttle needs to collect electrons from the lithiated graphite through the SEI layer. A large amount of heat is generated when the redox shuttle is activated to provide overcharge protection for lithium-ion batteries [20] . However, the potential impact of the heat generation on the cell has not been well studied. 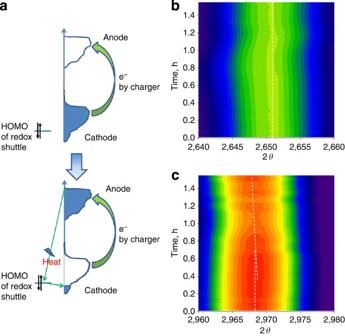Figure 6: Schematic energy diagram andin situHEXRD profiles. (a) Schematic energy diagram illustrating the potential heat generation at the anode side.In situHEXRD profiles of a Li4Ti5O4/LiMn2O4cell during overcharge test showing the lattice variation of (b) Al and (c) Cu. The electrolyte was 0.4 M Li2B12F9H3in EC/EMC (3:7, by weight). The current was 0.2 A (~1 C). Figure 6a shows a schematic energy diagram illustrating the potential impact of this heat generation. In general, under normal conditions, the energy level of the electrons in the anode is higher than that in the cathode, and the energy level of the highest occupied molecular orbital (HOMO) of the redox shuttle is lower than that of the electrons in the cathode. During normal charge, the external charger keeps pumping electrons from the cathode to the anode ( Fig. 6a , top). The redox shuttle remains inactive, as the energy level of its HOMO is still lower than that in the cathode. When the cell is overcharged, the electron level in the cathode is drained to a level below the HOMO of the redox shuttle, which then donates an electron to the cathode to prevent over draining of electrons from the cathode. The redox shuttle with singly occupied HOMO then diffuses to the anode and obtains an electron from the anode. Transferring electrons over the huge energy gap between the anode and the redox shuttle (~4.5 eV) leads to the generation of heat or breaking of chemical bonds at the anode side ( Fig. 7a , bottom). In addition, the energy released due to the electron transfer between the anode and the oxidized redox shuttle increases proportionally with the decrease of HOMO energy level, or increase of the redox potential, of the redox shuttle. Therefore, Li 2 B 12 F 12 is expected to release more heat than Li 2 B 12 F 9 H 3 when redox mechanism is activated. Figure 6: Schematic energy diagram and in situ HEXRD profiles. ( a ) Schematic energy diagram illustrating the potential heat generation at the anode side. In situ HEXRD profiles of a Li 4 Ti 5 O 4 /LiMn 2 O 4 cell during overcharge test showing the lattice variation of ( b ) Al and ( c ) Cu. The electrolyte was 0.4 M Li 2 B 12 F 9 H 3 in EC/EMC (3:7, by weight). The current was 0.2 A (~1 C). 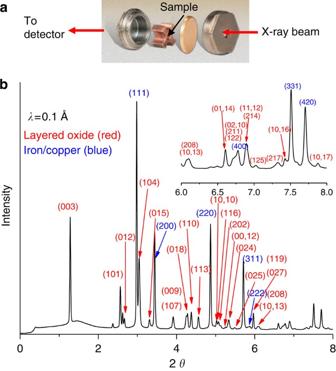Figure 7: Typical sample forin situHEXRD experiment to investigate the thermal stability of delithiated Li1-x[Ni1/3Mn1/3Co1/3]0.9O2. (a) Image of a stainless-steel high-pressure DSC sample holder for thermal-ramping experiment. (b) HEXRD pattern of a DSC sample containing about 1.5 mg delithiated Li1-x[Ni1/3Mn1/3Co1/3]0.9O2and about 1.5 μl nonaqueous electrolyte. The XRD pattern can be successfully indexed using two sets of cell parameters: one is the diffraction pattern of the layer oxide structure (space group 166, R-3mH) and the other is the cubic structure of stainless steel or copper (space group 225, Fm-3m). Full size image Figure 7: Typical sample for in situ HEXRD experiment to investigate the thermal stability of delithiated Li 1- x [Ni 1/3 Mn 1/3 Co 1/3 ] 0.9 O 2 . ( a ) Image of a stainless-steel high-pressure DSC sample holder for thermal-ramping experiment. ( b ) HEXRD pattern of a DSC sample containing about 1.5 mg delithiated Li 1- x [Ni 1/3 Mn 1/3 Co 1/3 ] 0.9 O 2 and about 1.5 μl nonaqueous electrolyte. The XRD pattern can be successfully indexed using two sets of cell parameters: one is the diffraction pattern of the layer oxide structure (space group 166, R-3mH) and the other is the cubic structure of stainless steel or copper (space group 225, Fm-3m). Full size image To validate this mechanism, we prepared a 180-mAh pouch cell using LiMn 2 O 4 as the cathode and Li 4 Ti 5 O 12 as the anode. The electrolyte was 0.4 M Li 2 B 12 F 9 H 3 in EC/EMC (3:7, by weight). After being charged/discharged for two cycles between 1.5 V and 2.8 V using a constant current of 0.2 A, the cell was continuously charged at a constant current of 0.2 A for 90 min, leading to about 50% overcharge. During this test, HEXRD profiles of the pouch cell were continuously collected at a rate of one spectrum per 20 s (see Supplementary Fig. S4 for full patterns and indexes of peaks). Figure 6b shows a contour plot of spectra around the (111) peak of aluminium between 2.64° and 2.66°. It can be seen that the lattice parameter of aluminium did not change throughout the experiment. However, the (111) peak of copper shifted towards smaller angles when the cell was overcharged at about 0.8 h; this peak shift was caused by the thermal expansion of copper when the cell was overcharged ( Fig. 6c ). This finding confirms that the activation of the redox shuttle dumps a large amount of heat at the anode side and can lead to thermal decomposition of the conventional SEI layer, which decomposes at a temperature as low as 60 °C. Therefore, a thermally stable SEI layer such as that formed with LiDFOB is highly desirable to avoid the direct exposure of lithiated graphite to the electrolyte when the cell is repeatedly overcharged. Better tolerance towards thermal abuse In situ HEXRD experiments during thermal ramping were carried out to investigate the potential impact of the new electrolytes on the thermal stability of delithiated Li 1.1 [Ni 1/3 Mn 1/3 Co 1/3 ] 0.9 O 2 , the HEXRD profile of a sample housed in the stainless-steel high-pressure vessel was well indexed with the layered structure and is shown in Fig. 7 . 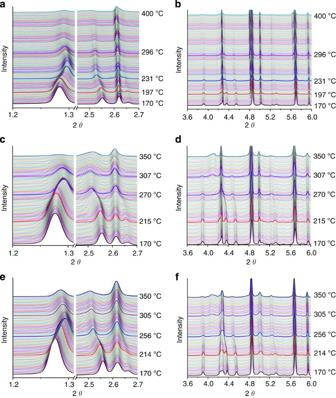Figure 8:In situHEXRD profiles of delithiated Li1-x[Ni1/3Mn1/3Co1/3]0.9O2during thermal abuse up to 400 °C. (a) Electrolyte of 1.2 M LiPF6in EC/EMC (3:7, by weight) and profile for a low 2θrange. (b) Same electrolyte as (a) but profile for a high 2θrange. (c) Electrolyte of 0.4 M Li2B12F12in EC/EMC (3:7, by weight) and profile for a low 2θrange. (d) Same electrolyte as (c) but profile for a high 2θrange. (e) Electrolyte of 0.4 M Li2B12F9H3in EC/EMC (3:7, by weight) and profile for a low 2θrange. (f) Same electrolyte as (c) but profile for a high 2θrange. Figure 8a show the in situ HEXRD profiles of delithiated Li 1.1 [Ni 1/3 Mn 1/3 Co 1/3 ] 0.9 O 2 in the presence of 1.2 M LiPF 6 in EC/EMC (3:7, by weight) and during thermal abuse from room temperature to 400 °C at a scanning rate of 5 °C min −1 . The delithiated electrode material was recovered from a Li/Li 1.1 [Ni 1.3 Co 1/3 Co 1/3 ] 0.9 O 2 coin cell that had been constant-voltage charged to 4.1 V. During the thermal abuse process, a phase transformation from a layered to spinel structure occurred at about 197 °C and finished at about 231 °C, after which the newly formed spinel phase decomposed. The phase transformation and decomposition of spinel phase resulted from the electrochemical/chemical reaction of the delithiated Li 1- x [Ni 1/3 Mn 1/3 Co 1/3 ] 0.9 O 2 and the nonaqueous electrolyte, which generated a large amount of heat. If this reaction were triggered in a lithium-ion battery, it could lead to the thermal runaway, causing a battery fire or even explosion. Therefore, a high onset temperature for these reactions is highly desired for the production of safer lithium-ion batteries. When LiPF 6 was replaced by Li 2 B 12 F 12 , the onset temperatures for these two reactions increased to 215 °C and 270 °C, respectively ( Fig. 8c ), due to the lack of HF in the electrolyte, which is believed to promote the thermal decomposition of delithiated cathodes [21] . Similar observation was also obtained for the sample using Li 2 B 12 F 9 H 3 -based electrolyte, the onset temperature for the interested reactions was 214 °C and 256 °C, respectively ( Fig. 8e ). Figure 8: In situ HEXRD profiles of delithiated Li 1- x [Ni 1/3 Mn 1/3 Co 1/3 ] 0.9 O 2 during thermal abuse up to 400 °C. ( a ) Electrolyte of 1.2 M LiPF 6 in EC/EMC (3:7, by weight) and profile for a low 2 θ range. ( b ) Same electrolyte as ( a ) but profile for a high 2 θ range. ( c ) Electrolyte of 0.4 M Li 2 B 12 F 12 in EC/EMC (3:7, by weight) and profile for a low 2 θ range. ( d ) Same electrolyte as ( c ) but profile for a high 2 θ range. ( e ) Electrolyte of 0.4 M Li 2 B 12 F 9 H 3 in EC/EMC (3:7, by weight) and profile for a low 2 θ range. ( f ) Same electrolyte as ( c ) but profile for a high 2 θ range. Full size image We have demonstrated that Li 2 B 12 F 12- x H x -based electrolytes possess several advantages over conventional LiPF 6 -based electrolyte. Graphite/Li 1.1 [Ni 1/3 Mn 1/3 Co 1/3 ] 0.9 O 2 cells using Li 2 B 12 F 9 H 3 -based electrolyte, using lithium difluoro(oxalato)borate as the electrolyte additive, maintained 70% capacity retention after being cycled at 55 °C for 1,200 cycles. In addition, the cells had excellent tolerance to low-rate continuous overcharge and high-rate pulse overcharge. Moreover, the Li 2 B 12 F 12- x H x -based electrolytes also improved the thermal stability of delithiated Li 1- x [Ni 1/3 Mn 1/3 Co 1/3 ] 0.9 O 2 cathodes. Therefore, we believe that Li 2 B 12 F 12- x H x -based electrolytes are promising for high performance and safe lithium-ion batteries designed for automobile and grid applications. In situ HEXRD during thermal abuse The experimental set-up for the in situ experiment was similar to that previously reported for solid-state synthesis [22] . A differential scanning calorimetry sample was placed vertically in a stainless-steel high-pressure vessel that was programmable thermally, and it was heated up to 400 °C at a constant heating rate of 5 °C per minute. During the course of thermal ramping, a high-energy X-ray hit the sample horizontally, and a PerkinElmer area X-ray detector collected the XRD patterns in the transmission geometry at a speed of 1 spectrum per 20 s. The XRD experiment was carried out at beamline 11-ID-C of the Advanced Photon Source of Argonne National Laboratory; the X-ray wavelength was 0.10804 Å. The collected 2D pattern was then integrated into conventional 1D data (intensity versus 2 θ ) using the fit2d programme [23] . In situ HEXRD during overcharge A Li 4 Ti 5 O 12 /LiMn 2 O 4 lithium-ion pouch cell was assembled using 0.4 M Li 2 B 12 F 9 H 3 in EC/EMC (3:7 by weight) as the electrolyte. The cell was first charged/discharged between 1.5 V and 2.8 V using a constant current of 0.2 A for two cycles. The initial capacity of the cell was about 0.18 Ah. Then, the cell was constant-current charged at 0.2 A for 90 min in the high-energy X-ray beam at beamline 11-ID-C of the Advanced Photon Source. The XRD patterns of the cell were collected every 20 s. Cycle-life characterization Cycle-life testing was conducted with both coin cells (1.6 mAh) and pouch cells (250 mAh) using graphite as the anode and Li 1.1 [Ni 1/3 Mn 1/3 Co 1/3 ] 0.9 O 2 as the cathode. The cells were first charged/discharged between 3.0 V and 4.1 V at a constant current of C/10 for two cycles. The cells were then cycled at either room temperature or 55 °C between 2.5 V and 4.1 V with a constant current of C/3. Low-rate continuous overcharge test This test was conducted with graphite/Li 1.1 [Ni 1/3 Mn 1/3 Co 1/3 ] 0.9 O 2 coin cells (about 1.6 mAh). The cells were periodically overcharged by charging the cell at a C/3 rate for 4 h with a voltage cutoff at 4.95 V, whichever was reached first, before constant-current discharging the cell to 3.0 V at C/3. High-rate pulse overcharge test For this test, graphite/Li 1.1 [Ni 1/3 Mn 1/3 Co 1/3 ] 0.9 O 2 coin cells (~1.6 mAh) were initially charged/discharged between 3.0 V and 4.1 V with a constant current of C/10 for two cycles before being constantly charged to 4.1 V. Then, the cells were periodically charged with a constant current of 20 mA (~12 C) for 18 s before resting for 1 h. The test stopped when 100 pulses were applied or when the upper voltage reached 4.95 V. This special testing procedure was adopted to mimic the hybrid pulse power characteristics test commonly used for hybrid electric vehicle batteries. Cyclic voltammetry Cyclic voltammograms of the Li 2 B 12 H 12− x F x -containing electrolytes were collected with a BAS-Zahner IM6 impedance analyser and a Li/Li/Pt three-electrode cell at a scanning rate of 10 mV s −1 . The diameter of the Pt-working electrode was about 1 mm. Cyclic voltammetry was performed in an argon-filled glove box. Ab initio calculations All the calculations reported in this work were carried out with the Gaussian03 computational package [24] . Hartree–Fock theory with a basis set of 6-31G+(d, p) [HF/6-31G+(d,p)] was used for full geometry optimization. Karl Fisher measurement Moisture titration was performed with an Orion Model AF7 Coulometric Karl Fischer titrator, using Hydranal Coulomat AF7 anolyte and Hydranal Coulomat CG-K catholyte. The electrolyte samples were stored and handled in an argon glove box. Each sample was titrated at least twice. The values reported are given in ppm by weight of H 2 O in the electrolyte. HF titration HF acid titration was performed with a 5-ml glass burette with graduations of 0.01 ml using a 0.02 N sodium hydroxide (NaOH) aqueous solution. The pH indicator was bromothymol blue (0.04 wt% in water), which is yellow at pH <6 and blue at pH >7. A dry polypropylene syringe (1 ml size) and polypropylene Erlenmeyer flask (50 ml) were used when handling electrolyte samples to prevent the reaction of glass with possible HF acid. This titration technique was done by first placing ~3 ml of crushed ice (pH neutral) in the plastic Erlenmeyer flask with ~1 ml of pH-neutral water and a couple of drops of indicator. Approximately 0.2 ml of electrolyte was drawn into the plastic syringe, weighed to 0.1 mg accuracy and expelled onto the ice slurry. The flask was swirled while the NaOH solution was carefully metered out through the burette. Addition of the NaOH drops was stopped immediately when the slurry colour turned to a slight blue tint (from yellow). If after 30 s, the colour returned to yellow, more NaOH was added (usually one or two additional drops was enough). Note that the colour will eventually turn yellow again if time is allowed to pass or if the slurry warms up. This titration was done as quickly as possible to make sure that ice remained present in the slurry. The empty syringe was then weighed to obtain the electrolyte sample weight. The acid level was easily calculated with the assumption that it was pure HF. Each sample was titrated at least twice. The values reported are given in ppm by weight of HF in electrolyte. How to cite this article: Chen, Z. et al . New class of nonaqueous electrolytes for long-life and safe lithium-ion batteries. Nat. Commun. 4:1513 doi: 10.1038/ncomms2518 (2013).